A route for a strong increase of critical current in nanostrained iron-based superconductors The critical temperature T c and the critical current density J c determine the limits to large-scale superconductor applications. Superconductivity emerges at T c . The practical current-carrying capability, measured by J c , is the ability of defects in superconductors to pin the magnetic vortices, and that may reduce T c . Simultaneous increase of T c and J c in superconductors is desirable but very difficult to realize. Here we demonstrate a route to raise both T c and J c together in iron-based superconductors. By using low-energy proton irradiation, we create cascade defects in FeSe 0.5 Te 0.5 films. T c is enhanced due to the nanoscale compressive strain and proximity effect, whereas J c is doubled under zero field at 4.2 K through strong vortex pinning by the cascade defects and surrounding nanoscale strain. At 12 K and above 15 T, one order of magnitude of J c enhancement is achieved in both parallel and perpendicular magnetic fields to the film surface. Superconductor’s lossless current flow enables the design of highly dense and compact equipment, and hence offers powerful opportunities for increasing the capacity and the efficiency of power grids [1] , [2] . Superconducting coils use magnetic fields to store energy with near zero energy loss and can power drive rotary machines. Three properties of superconductors important for energy applications are superconducting transition temperature (also known as critical temperature) T c , upper critical field, and electrical current-carrying capacity. They arise from different aspects of the superconducting states. T c is directly related to the mechanism of superconductivity. The superconducting state emerges at T c from interactions between electrons that form the Cooper pairs. The upper critical field, H c2 , is the highest magnetic field at which superconductivity is finally suppressed. In contrast to T c and H c2 , the current-carrying capacity, measured by the practical critical current density J c , is governed by the vortex pinning strength, which is determined by the ability of defects in superconducting materials to pin the vortices carrying magnetic flux. Defects create local regions with depressed pairing potential, which can pin the vortices. By doing so, unfortunately, defects tend to preclude the Cooper pair formation and hence drive down the T c of cuprates and iron-based superconductors with short coherence lengths. It is a very difficult and challenging task to raise T c and J c simultaneously by means of introducing defects in the same cuprates and iron-based superconducting materials. Tremendous efforts have been made so far to optimize the defects landscape, to enhance J c , while keeping the degradation of T c to a minimum in cuprates and iron-based superconductors. Indeed, great improvements in J c have been obtained in cuprate and in iron-based superconducting films as well, by introducing artificially designed defects such as precipitate and columnar defects, but at the cost of T c degradation [3] , [4] , [5] , [6] , [7] , [8] , [9] , [10] . Iron-based superconductors [11] have attracted much attention in potential high-field applications due to their relatively high T c , high H c2 , and small anisotropy γ [12] , [13] . Recent reports show that high-quality epitaxial films have been grown on single crystal substrates, mostly used for exploring the fundamental properties of iron-based superconductors [8] , [9] , [10] , [14] , [15] , [16] , [17] , [18] . We have reported very high- J c FeSe 0.5 Te 0.5 (FST) films with CeO 2 buffer layer on single crystals and a metal substrate of coated conductors [16] . We found that further J c improvement by controlled growth of pinning defects, in the iron-based superconducting films we processed, is becoming increasingly difficult. This motivated us to look for alternative routes. Ion irradiation is a well-established method for artificially introducing various defects into superconducting materials in a fairly predictable and controllable manner by choosing appropriate ion species and energy [3] , [19] , [20] , [21] , [22] . Transmission electron microscopy (TEM) cross-sectional images along the ion traces in 230 MeV Au-irradiated Bi 2 Sr 2 CaCu 2 O x single crystals showed several types of morphology of defects from parallel columnar defects to disordered cascade defects, as the ion energy is decreased in the crystals [22] . It is also well known that light ion irradiations produce smaller damaged volume fractions in the target materials than heavy ion irradiation and requires a much higher dosage to produce enough defects for flux pinning because of the significantly large ionization loss. These defects produced by ion irradiation would account for the depression of T c in YBa 2 Cu 3 O y (YBCO), which is proportional to the average number of defects [23] . Recently, a low-energy ion irradiation has been revisited and suggested as a practically feasible approach to improve flux pinning in YBCO [24] , [25] , [26] . In single crystals of iron-based superconductors, it has been found that ion irradiations, as a whole, improve J c and its J c enhancements persist up to much higher fluencies than in cuprate superconductors, although T c is suppressed with increasing irradiation doses [27] , [28] , [29] . In contrast, the irradiated iron-based superconducting films have not shown as positive effects as found in single crystals [30] , [31] . It is clear that the key to the enhancement of J c in superconductors is in the design of defect landscape that must be tailored to a superconductors’ chemistry, crystal structure, and materials’ geometric aspect. Here we show a strategy on nanostructure control in iron-chalcogenide superconducting FST films with low-energy proton irradiation. Through extensive TEM characterization, we found nanoscale strain modulations in FST films irradiated with 1 × 10 15 p cm –2 dose of 190 keV proton. Enhanced from 18.0 to 18.5 K is observed in the irradiated films due to the nanoscale compressive strain and proximity effect. The low-energy proton irradiation also yields self-field J c enhancement from 0.9 MA cm –2 up to 1.4 MA cm –2 at 4.2 K. The cascade defects and nanoscale strain produced by low-energy proton irradiation are found to provide strong vortex pinning, resulting in remarkable enhancements of J c at both zero field and high magnetic field in all temperatures, and high maximum pinning force F p,max of ∼ 120 GN m –3 for H // ab at 27 T and 4.2 K. 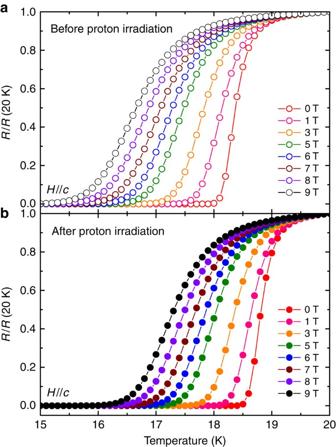Figure 1: Temperature dependence of normalized resistivity. ρ(T)/ρ(20 K) at 0–9 T//cfor the FST film before (a) and after (b) 190 keV proton irradiation with 1 × 1015p cm−2dose. Transition temperature and microstructural analysis Figure 1a,b show the temperature dependence of the normalized resistivity up to 9 T with H // c for the FST film before and after 190 keV proton irradiation at 1 × 10 15 p cm −2 fluence, respectively. We determine the and the irreversibility field ( H irr ) using 0.01 ρ n criteria and H c2 using 0.9 ρ n criteria with ρ n = ρ (20 K). As previously reported [16] , the CeO 2 -buffered FST film (pristine film) exhibits enhanced =18.0 K, which is ∼ 30% higher than that found in the bulk materials [32] . Strikingly, we found that the irradiated FST film does not show any T c degradation, rather an increase of T c by ∼ 0.5 K. The enhancement of T c by irradiations, with either light ion or heavy ion, was not known in iron-based superconductors previously [27] , [28] , [29] , [30] , [31] . Figure 1: Temperature dependence of normalized resistivity. ρ ( T )/ ρ (20 K) at 0–9 T// c for the FST film before ( a ) and after ( b ) 190 keV proton irradiation with 1 × 10 15 p cm −2 dose. Full size image In iron-chalcogenide superconductors, there have been many reports on enhancement of T c for bulk materials [33] , [34] , [35] , [36] , [37] , wires [38] and films [16] , [39] , [40] , [41] , [42] , [43] , [44] . Possible explanations can be grouped into three categories so far: (1) an interface effect, (2) an elimination of the influence of excess Fe at the interstitial sites of the Te/Se(S) layer and (3) a strain effect. The first group is based on the observation of monolayer FeSe films on SrTiO 3 substrate [39] , [40] . The enhanced superconductivity is generally believed to be the result of the interface between two very different materials and not relevant to our FST film of ∼ 100 nm thick. The second group is based on the post-annealing effect [35] , [36] , [37] . This could be attributed to a reduction of excess Fe, which creates magnetic moments and causes pair breaking [45] . The reasonable concern could be raised that the enhancement of T c in the proton-irradiated FST films is due to the suppression of the influence of excess Fe. To address this concern, we performed extensive high-resolution TEM (HRTEM) and scanning TEM (STEM) with high-angle annular dark field detector (HAADF) characterization. 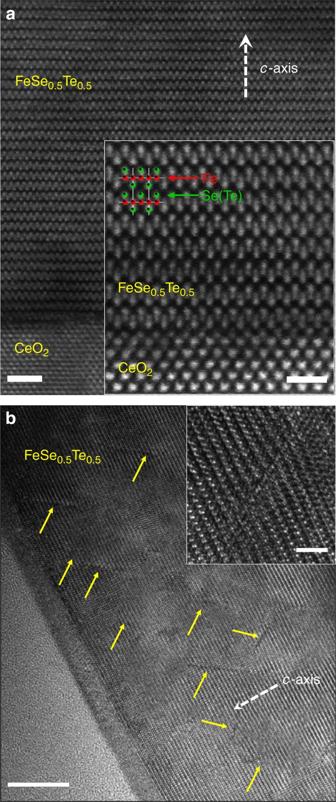Figure 2: Microstructure of FST films. (a) STEM-HAADF images of the representative FST film on the CeO2buffer layer. Scale bar, 2 nm. Inset: high-resolution image at the interface between CeO2and FST. Scale bar, 1 nm. (b) HRTEM image of FST film irradiated with 190 keV proton. Scale bar, 10 nm. Inset: high-resolution image of splayed cascade defect and strain field produced by 190 keV proton irradiation. Scale bar, 2 nm. Figure 2a displays representative STEM–HAADF image of the pristine FST film. The FST film is epitaxially grown on the CeO 2 buffer layer. STEM–HAADF image also reveals the very sharp FST-CeO 2 interface without the chemical reaction layer reported in FST/CaF 2 interface [42] . What is more remarkable here is that excess Fe, which is supposed to occupy the interstitial site in many iron-chalcogenide bulk samples, is not present in the FST film. Note: the presence of excess Fe in the interstitial sites is one of the major issues in iron chalcogenide superconductor, which lowers H c2 . The absence of excess Fe in our FST films deposited by pulsed laser deposition method is consistent with the observation that these FST films retain excellent performance at high field [15] , [16] , [46] . This is of great advantage for high-field applications. Figure 2: Microstructure of FST films. ( a ) STEM-HAADF images of the representative FST film on the CeO 2 buffer layer. Scale bar, 2 nm. Inset: high-resolution image at the interface between CeO 2 and FST. Scale bar, 1 nm. ( b ) HRTEM image of FST film irradiated with 190 keV proton. Scale bar, 10 nm. Inset: high-resolution image of splayed cascade defect and strain field produced by 190 keV proton irradiation. Scale bar, 2 nm. Full size image The third group is related to the strain effect on T c (refs 33 , 34 , 38 ), especially in iron-chalcogenide superconducting films [16] , [41] , [42] , [43] , [44] . Figure 2b shows a cross-sectional HRTEM image of the FST film irradiated with 190 keV proton. We observed splayed cascade defects produced by proton irradiation over the entire film. An enlarged view of a typical defect is displayed in the inset. The stopping range of ions in matter model [47] predicts that with increasing depth in Al foil covered on the FST film ( Supplementary Fig. 1 ), the angle distribution of the proton broadens, producing an angular splay for the proton. Previously, disordered spherical cascade defects were found to exist in the low-energy region of the Bi 2 Sr 2 CaCu 2 O x crystals [22] . Given that nuclear scattering events produce angular deviations from the original incident angle as the incident ions proceed through a target material, it is not surprising that light mass proton with a low energy of 190 keV easily tilted away from the original incident angle (0°) and create the disordered cascade defects. According to Anderson’s theorem [48] , the T c and the superconducting density of states in conventional s -wave superconductors are not affected by the non-magnetic impurity created by proton irradiation, whereas non-magnetic impurities can act as strong scattering centres and suppress T c by pair breaking in d -wave [49] or s ± wave [50] superconductors. In striking contrast, here we observed enhanced T c in the FST films after proton irradiation. Now we propose another mechanism to explain the enhancement of T c by proton irradiation. We note that besides the clearly visible cascade, there is also a curvature of the lattice fringe inwardly directed, which produces strain field around the cascade defect. Similar strain fields created by low-energy proton and neutron irradiation were observed in YBCO single crystals from a previous TEM study [51] , [52] . Although the size of the cascade defects is about 1 ∼ 2 nm in diameter and ∼ 10 nm wide, the strain fields are expected to extend far out to the cascade defect, especially in the radial direction and, as a result, can cause the local lattice distortion. Origin of enhanced T c and nanoscale lattice strain To see the cascade defect induced local lattice distortion, we Fourier transform two circled areas I and II in Fig. 3a , to get the diffractogram of the area of interest, as shown in the inset I and II. Intensity profiles from the central spot (000) to the reflection spots is then obtained for the measurement and the comparison of the positions of the reflection spots, as shown in Fig. 3b . The position of the 002 spot from circle I (green line) just slightly shift to the left in comparison with that from the circle II (black line), indicative of almost same c -lattice parameter in the irradiated FST film. On the other hand, the position of the 100 peak from local area I and II are not the same, indicative of large lattice variation along a axis parameter. We can calculate the strain map by geometrical phase analysis [53] , [54] , [55] . 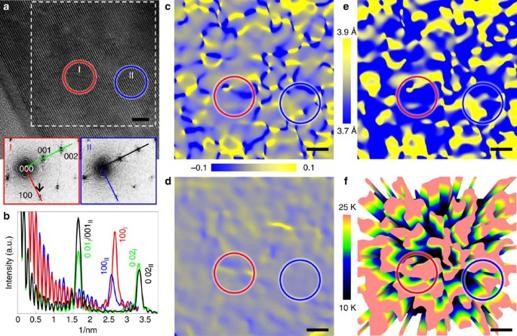Figure 3: Strain analysis in a 190 keV proton irradiated FST film. (a) HRTEM image. The inset I and II are the diffractogram from the circled area I (red) and II (blue), respectively. (b) Intensity line profiles of 001/002 (green and black) and 100 (red and blue) spots from the scan lines shown in the inset I and II ofa. (c,d) Strain maps of in-planeɛxx(c) and out-of-planeɛzz(d) calculated by geometrical phase analysis (GPA)53,54,55from the square area outlined by dash line ina. The colour bar in the middle indicates the strain from −0.1 (compressive) to 0.1 (tensile). (e) Map of in-plane lattice parameter determined from the GPA map inc. The colour bar in the left indicates the change in lattice parameter from 3.7 to 3.9 Å. (f) Perspective view of the spatial distribution ofTccalculated from the local strain (Supplementary Fig. 3). The red and blue circles show the same area. Scale bar, 5 nm (a,c–f). Figure 3c,d show the in-plane ɛ xx ( a axis direction) and the out-of-plane ɛ zz ( c axis direction) maps retrieved from the square area marked by the dash line in Fig. 3a . The averaged a - and c -lattice parameters were determined to be 3.77 and 5.95 Å, respectively, from the diffractogram of the whole image. The map of ɛ xx ( Fig. 3c ) shows extreme spatial variation of strains. Deep valleys (blue) are the highly compressed region with compressive strain ɛ xx ≅ −0.1, whereas sharp peaks (yellow) are the highly stretched region with tensile strain ɛ xx ≅ 0.1. These two extreme domains are nanoscopically entangled with each other in the irradiated FST film. This is in striking contrast to the map of ɛ zz in Fig. 3d , which is dominated by large interconnected areas of weak, strained areas. In contrast to the large strain observed in the irradiated FST film, the unirradiated FST film shows little strain in both in-plane ɛ xx and out-of-plane ɛ zz ( Supplementary Fig. 2 ). From the ɛ xx in the irradiated FST film, we can calculate lattice parameter map: a = a 0 (1+ ɛ xx ), where a 0 is the lattice parameter from the reference area (solid blue circle in Fig. 3a ). The result is shown in Fig. 3e . We noticed that low-energy proton irradiation causes more than 5% variation in lattice parameter a ranging from 3.7 to 3.9 Å over merely a few nanometre scale randomly distributed in the FST films. Red circles in Fig. 3a–f show the same area containing one cascade defect. Under electron, neutron or ion irradiation, point defect clusters are also produced in the form of vacancy and interstitial clusters from collision cascade defects in irradiated materials [20] , [21] , [51] , [52] . These clusters could cause the great compression-–tension strain fields at a nanoscale alongside the cascade defects. Figure 3: Strain analysis in a 190 keV proton irradiated FST film. ( a ) HRTEM image. The inset I and II are the diffractogram from the circled area I (red) and II (blue), respectively. ( b ) Intensity line profiles of 001/002 (green and black) and 100 (red and blue) spots from the scan lines shown in the inset I and II of a . ( c , d ) Strain maps of in-plane ɛ xx ( c ) and out-of-plane ɛ zz ( d ) calculated by geometrical phase analysis (GPA) [53] , [54] , [55] from the square area outlined by dash line in a . The colour bar in the middle indicates the strain from −0.1 (compressive) to 0.1 (tensile). ( e ) Map of in-plane lattice parameter determined from the GPA map in c . The colour bar in the left indicates the change in lattice parameter from 3.7 to 3.9 Å. ( f ) Perspective view of the spatial distribution of T c calculated from the local strain ( Supplementary Fig. 3 ). The red and blue circles show the same area. Scale bar, 5 nm ( a , c – f ). Full size image It is well known that compressive strain, especially along the in-plane direction, plays a crucial role in enhancing T c in FST films [16] , [41] , [42] , [43] . Now, we attempt to correlate the strain and T c in the irradiated films quantitatively, based on the analysis given by Bellingeri et al . [41] , that a axis lattice parameter is approximately linearly proportional to T c . A three-dimensional false-colour image in Fig. 3f shows the spatial variation of T c obtained by using the linear relation given by Bellingeri et al . [41] ( Supplementary Fig. 3 ). High- T c (highly compressive) and low- T c (highly tensile) regions are linked in a network similar to a cobweb in the irradiated FST films, with the highest T c reaching ∼ 25 K and the lowest T c reaching ∼ 15 K. The enhanced T c regions in the irradiated FST film rises from these contracted lattice parameter domains (highly compressive strain region) that are just 5 nm apart in average. This distance is comparable to the superconducting coherence length of FeSe 1– x Te x (0.5< x <0.85), estimated to be around 2.6 nm at zero temperature using the Ginzburg–Landau theory [56] , [57] . The irradiated FST films consist of small puddles of different T c values as shown in Fig. 3f . Proximity effect should lead to near homogeneous T c ( ∼ 18 K) in the film as a whole. There is greater volume associated with the compressive strain in a axis direction than that with tensile strain in the irradiated FST films, resulting in the higher value of T c as demonstrated in Fig. 1 . Irreversibility field and upper critical field Now, we turn our attention to vortex pinning behaviour in the irradiated FST films. 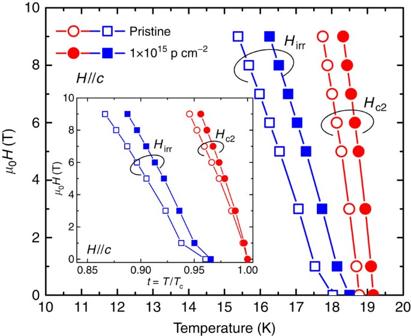Figure 4: Upper critical field and irreversibility field. Upper critical fieldHc2(T) and irreversible fieldHirr(T) (H//c) as a function of temperature up to 9 T//cfor FST films before and after proton irradiation determined fromFig. 1. Inset: normalized temperature (t=T/Tc) dependence ofHc2andHirrfor the same field orientation. Error bars are of a size smaller than the data points. Figure 4 shows the temperature dependence of irreversibility field H irr and H c2 for H // c . Both H irr and H c2 shift to higher T for the proton-irradiated film. When plotted as a function of t = T / T c , H irr and H c2 increase after proton irradiation can be compared. We found the increase in H irr is even more significant and produces a larger pinned vortex region, which suggests the cascade defects are strong pinning centres [20] , [21] , [58] . This is particularly important for the potential applications of the iron-based superconductor, as it can be operated in a larger-phase space. Figure 4: Upper critical field and irreversibility field. Upper critical field H c2 ( T ) and irreversible field H irr ( T ) ( H // c ) as a function of temperature up to 9 T// c for FST films before and after proton irradiation determined from Fig. 1 . Inset: normalized temperature ( t = T/T c ) dependence of H c2 and H irr for the same field orientation. Error bars are of a size smaller than the data points. Full size image J c in high magnetic field up to 34.5 T Strong enhancement of J c is shown in Fig. 5a , where we plot J c ( H ) for H // c at 4.2 K for 190 keV proton irradiation. The irradiated FST film has a larger self- and in-field J c than the pristine film. The self-field J c enhances from 0.9 MA cm –2 up to 1.4 MA cm –2 . Normalized J c ( H ) dependence of the FST films before and after irradiation is shown in a log–log pot in Fig. 5b . The regime of a nearly constant J c up to a characteristic crossover field of B * (90% of normalized J c ( H )), is associated with a single vortex pinning regime, followed by a rollover to a power-law regime ( J c ∝ B – α ) at intermediate fields, at which vortex–vortex interactions become relevant and a collective pinning vortex motion is dominant. We found that the pristine FST film already has high B * of 0.26 T, which is higher than BaFe 2 As 2 :P+BaZrO 3 films [8] . After proton irradiation, B * in the FST film increases up to 0.40 T. Studies by Dam et al . [59] showed that no correlation is found between the density of linear defects and the value of J c in the single vortex-pinning regime. The ratio between B *’s before and after irradiation is almost the same as the one between self-field J c ’s. Thus, the increase in B * after irradiation might just come from the increase in the self-field J c . At intermediate field, however, J c ( H ) in both FST films does not follow a power-law decay, although we observe a roundish J c dependence with magnetic field, as shown in Fig. 5b . The similar behaviour, that is, the absence of a power-law decay (or almost no change in α ), has been found in both cuprate and iron-based superconducting films with strong vortex pinning [6] , [7] , [8] , [60] . It appears the irradiated FST films also exhibit an extremely good J c retention at low field, indicating the potential of the iron-based superconductors for utility cable application. 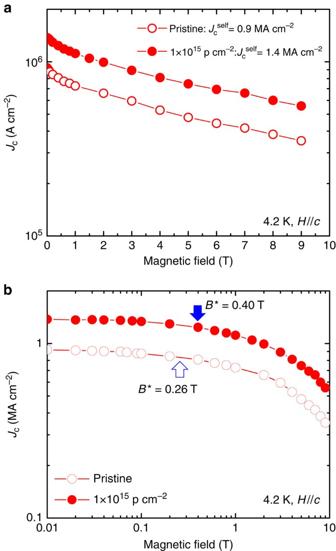Figure 5: Critical current density as a function of magnetic fields up to 9 T. (a)Jc(H//c) for the FST film before and after 190 keV proton irradiation with 1 × 1015p cm−2dose at 4.2 K. (b) Same data plotted in log-log scale. The arrows indicate the field of the crossover fieldB*. Figure 5: Critical current density as a function of magnetic fields up to 9 T. ( a ) J c ( H // c ) for the FST film before and after 190 keV proton irradiation with 1 × 10 15 p cm −2 dose at 4.2 K. ( b ) Same data plotted in log-log scale. The arrows indicate the field of the crossover field B *. 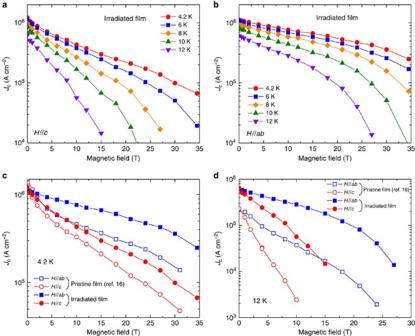Figure 6: High-field critical current density up to 34.5 T. (a,b)Jc(H) for proton-irradiated FST film with 1 × 1015p cm−2dose at different temperature up to 34.5 T withH//candH//ab, respectively. (c,d)Jc(H) for the irradiated FST film up to 34.5 T compared with the pristine FST film16at 4.2 and 12 K, respectively. Full size image High-magnetic field transport measurement of the irradiated FST film was performed up to 34.5 T. Figure 6a,b show J c ( H ) at various temperatures for H // c and H // ab , respectively. In Fig. 6c,d , we plot J c ( H ) for the irradiated FST film at 4.2 and 12 K, together with the J c ( H ) data taken on the pristine film [16] for comparison. The irradiated FST film clearly has a much better field performance for both H // ab and H // c . We found the J c at 12 K increased by one order of magnitude after irradiation over 15 T for H // ab and over 6 T for H // c . Enhancement of vortex pinning at higher temperature (12 K) is much more significant compared with that at low temperature (4.2 K). Figure 6: High-field critical current density up to 34.5 T. ( a , b ) J c ( H ) for proton-irradiated FST film with 1 × 10 15 p cm −2 dose at different temperature up to 34.5 T with H // c and H // ab , respectively. ( c , d ) J c ( H ) for the irradiated FST film up to 34.5 T compared with the pristine FST film [16] at 4.2 and 12 K, respectively. Full size image Vortex-pinning properties The effect of cascade defects and strain modulation from proton irradiation on vortex pinning properties can be appreciated by evaluating the pinning force F p = J c × μ 0 H . 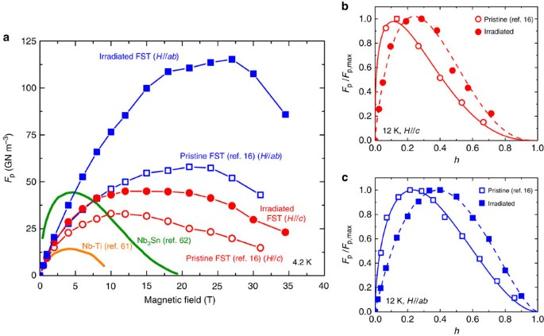Figure 7: High-field pinning force. (a)Fp(H) for FST film before and after 190 keV proton irradiation with 1 × 1015p cm−2dose at 4.2 K, compared with NbTi (ref.61) and Nb3Sn (ref.62) wires. (b,c) NormalizedFp(h) for FST film before (open symbols) and after (close symbols) proton irradiation at 12 K forH//candH//ab, respectively, whereas solid (before) and dashed (after) lines are the corresponding fitting curves. Figure 7a shows F p ( H ) for the pristine [16] and the irradiated FST films at 4.2 K together with the data for NbTi (ref. 61 ) and Nb 3 Sn (ref. 62 ) wires for comparison. After proton irradiation, the F p peak width broadens and the enhancement of F p is prominent in the high-field region for H // c . The maximum pinning force F p,max ∼ 45 GN m –3 , which is increased by ∼ 30%, occurs at 12 T in the irradiated FST film for H // c . At H // ab , a remarkably high F p,max of ∼ 120 GN m –3 is reached for the irradiated FST film at 27 T, that is, an enhancement of ∼ 200% over the pristine film. These results suggest that the cascade defects and nanoscale strain field can be highly effective pinning centres, especially for H // ab . Extensive researches by Llordés et al . [63] and Deutscher [64] have showed a similar result that the nanoscale strain present in ɛ zz map is responsible for a strong enhancement of pinning force for H // c . In the irradiated FST film, the nanoscale strain observed in ɛ xx map can lead to the extremely high F p,max and the shift of the F p,max to high field for H // ab . Figure 7: High-field pinning force. ( a ) F p ( H ) for FST film before and after 190 keV proton irradiation with 1 × 10 15 p cm −2 dose at 4.2 K, compared with NbTi (ref. 61 ) and Nb 3 Sn (ref. 62 ) wires. ( b , c ) Normalized F p ( h ) for FST film before (open symbols) and after (close symbols) proton irradiation at 12 K for H // c and H // ab , respectively, whereas solid (before) and dashed (after) lines are the corresponding fitting curves. Full size image The reduced pinning force density as a function of reduced magnetic field for the pristine [16] and the irradiated FST films at 12 K is plotted in Fig. 7b,c , respectively. Solid and dashed fitting lines are calculated using , where f p0 is a constant. The values of exponent fitting parameters p and q are given in the Supplementary Table 1 . After irradiation, we found that the exponent p increases significantly to 0.57 for H // c from 0.33 before the irradiation, whereas for H // ab , p increases to 0.97 (towards unity) from 0.85 before the irradiation. The exponent q decreases substantially to 1.87 ( H//c ) and 1.56 ( H // ab ) from the values of 2.63 ( H // c ) and 2.68 ( H // ab ) before the irradiation. It is perhaps instructive to compare our results with the vortex pinning for α -Ti ribbon in Nb-Ti wires, which shows that cold work reduces the dimensions of the α -Ti precipitates to optimum size for vortex pinning, resulting in the F p curve shape (refs 65 , 66 ). Of course, rigorous analysis and modelling would need to take into account of accurate information on the defect size, associated strain field and morphology/anisotropy, which is beyond the current studies. Nevertheless, both fitting parameters p and q are found approaching unity in the irradiated films, which is consistent with the structural observation shown in Fig. 3 . The cascade defect and nanoscale strain act more or less similar to elongated point-defect pinning. The scaling behaviour for H // ab of the irradiated FST film may be attributed to strong vortex pinning due to a dense array of nanoscale cascade defect and longer extension of the strain field along the a axis direction. In conclusion, a robust enhancement of T c and J c has been realized simultaneously in the FST film irradiated with 1 × 10 15 p cm –2 dose of 190 keV proton, resulting in an increase of from 18.0 to 18.5 K and a self-field J c enhancement from 0.9 MA cm –2 up to 1.4 MA cm –2 at 4.2 K. TEM structural characterization provides direct atomic-scale imaging of the collision cascade defects and the surrounding strain field, produced by low-energy proton irradiation. The highly compressive strain increases T c of the irradiated films through the proximity effect. The cascade defects and nanoscale strain are found to provide strong vortex pinning, leading to the increase of J c by one order of magnitude at 12 K over 6 T and record high F p,max of ∼ 120 GN m –3 for H // ab at 27 T and 4.2 K. This study demonstrates that it is possible to achieve significant enhancement of J c without T c reduction through the design of vortex pinning landscape that takes advantage of cascade defects and associated strain field. Further improvement of the performance of these films can be expected with fine tuning of the morphology of defects and strain configuration. The low-energy ion sources are inexpensive to operate and are readily available commercially. This route provides a practical solution to the central limiting factor that controls the performance of superconducting wires and tapes that underpins all superconducting applications. Sample preparation FST films of 100–130 nm thickness are grown by pulsed laser deposition with CeO 2 buffer layer on SrTiO 3 single-crystalline substrates [15] , [16] , [46] . The FST films characterized in advance were covered by 1.5 μm thick Al foil and irradiated with 190 keV protons at dose of 1 × 10 15 p cm –2 ( Supplementary Fig. 1 ). At this energy, the simulation using the stopping range of ions in matter code [47] shows that the stopping region (Bragg peak) of the protons is ∼ 100 nm from the FST film surface, which maximizes the effect of cascade defect creations in the FST films. Characterization Microstructures of the 190 keV proton-irradiated FST film were characterized using aberration-corrected STEM and HRTEM. All transport characterizations were performed on the same films before and after irradiation. Low-field measurements were performed by the standard four-probe method in a physical property measurement system (Quantum Design), whereas the high-field measurements were done in 35 T direct current magnet at National High Magnetic Field Laboratory in Tallahassee. Data availability All relevant data supporting the finding of this study are available within the article and its Supplementary Information file or available from the corresponding authors upon request, which should be addressed to T.O. and Q.L. How to cite this article: Ozaki, T. et al . A route for a strong increase of critical current in nanostrained iron-based superconductors. Nat. Commun. 7, 13036 doi: 10.1038/ncomms13036 (2016).